MEIOB exhibits single-stranded DNA-binding and exonuclease activities and is essential for meiotic recombination Meiotic recombination enables the reciprocal exchange of genetic material between parental homologous chromosomes, and ensures faithful chromosome segregation during meiosis in sexually reproducing organisms. This process relies on the complex interaction of DNA repair factors and many steps remain poorly understood in mammals. Here we report the identification of MEIOB, a meiosis-specific protein, in a proteomics screen for novel meiotic chromatin-associated proteins in mice. MEIOB contains an OB domain with homology to one of the RPA1 OB folds. MEIOB binds to single-stranded DNA and exhibits 3′–5′ exonuclease activity. MEIOB forms a complex with RPA and with SPATA22, and these three proteins co-localize in foci that are associated with meiotic chromosomes. Strikingly, chromatin localization and stability of MEIOB depends on SPATA22 and vice versa. Meiob- null mouse mutants exhibit a failure in meiosis and sterility in both sexes. Our results suggest that MEIOB is required for meiotic recombination and chromosomal synapsis. Meiosis, the hallmark of gametogenesis in sexually reproducing organisms, creates haploid germ cells from diploid progenitors and ensures their genetic diversity through recombination. Physical links between homologous chromosomes permit the formation of crossovers required for allele recombination and also facilitate accurate chromosome segregation at the first meiotic cell division [1] , [2] . Meiotic recombination is initiated at DNA double-strand breaks (DSBs) generated by SPO11 (ref. 3 ); these DSBs become resected from the 5′-end, yielding extended 3′-single-stranded DNA (ssDNA) overhangs [4] . Replication protein A (RPA) coats ssDNA, forming nucleoprotein filaments that prevent degradation and secondary structure formation. Subsequent invasion of the 3′-single strand into the duplex of the homologue is mediated by DMC1 and RAD51. Strand invasion causes the displacement of one strand of the homologue, resulting in D-loop formation [5] . The invading 3′-end primes new DNA synthesis, such that D-loop extension towards the second end allows for the capture of the 3′-ssDNA end of the other break (second end). End ligation leads to the formation of double Holliday junctions. Although early steps of meiotic recombination (DSB formation, end resection, strand invasion and D-loop formation) have been relatively well characterized, the intermediate steps of this process, such as second-end capture, are poorly defined. RPA is a conserved ssDNA-binding heterotrimer complex of RPA1, RPA2 and RPA3 (ref. 6 ). The four oligonucleotide-binding (OB) folds of RPA1 mediate ssDNA binding of the RPA complex [7] . RPA is essential for many aspects of DNA metabolism, notably DNA replication, DNA repair and meiotic recombination. During meiotic recombination, RPA binds to various ssDNA intermediates, including resected 3′-ssDNA and the D-loop. Studies of mutant alleles of yeast RPA1 have demonstrated that RPA is required for meiotic recombination [8] . RPA is indispensible for mouse development; a homozygous point mutation in Rpa1 causes early embryonic lethality [9] . Here we report the identification of meiosis-specific with OB domains (MEIOB), a meiosis-specific protein with homology to one OB fold of RPA1, in a systematic proteomics screen for meiotic chromatin-associated proteins. We find that mouse MEIOB has evolved to fulfill an essential function in meiosis. Proteomics screen for meiotic chromatin-associated proteins To systematically identify proteins that are associated with meiotic chromosomes, we isolated chromatin from postnatal day 18 (P18) testes, which lack post-meiotic germ cells and are thus highly enriched for meiotic germ cells. Our adaptation of a chromatin purification protocol for testis samples yielded highly pure chromatin ( Fig. 1a ) [10] , [11] . SYCP2, a synaptonemal complex protein associated with meiotic chromatin [12] , was present in the chromatin fraction, whereas the cytoplasmic germ cell-specific protein TEX19 was not detectable in the chromatin fraction by western blot analysis ( Fig. 1b ) [13] . To improve detection of proteins with low abundance, we separated chromatin-associated proteins from P18 testes by SDS–polyacrylamide gel electrophoresis (PAGE) and analysed ten different size fractions by tandem mass spectrometry (MS/MS; Fig. 1c ). A total of 1,300 proteins with at least one unique peptide were identified. 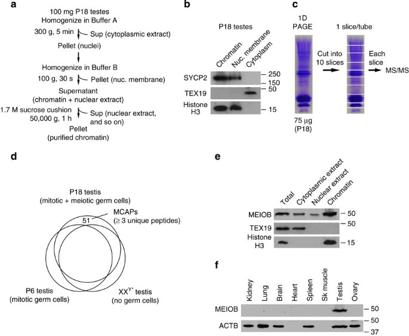Figure 1: Proteomic identification of meiotic chromatin-associated proteins from mouse testes. (a) Biochemical purification of chromatin from P18 testes. (b) Purity assessment of isolated meiotic chromatin by western blotting. SYCP2 is known to associate with meiotic chromatin. TEX19 is a cytoplasmic protein control. Histone H3 is a ubiquitous chromatin-associated protein. (c) Identification of chromatin-associated proteins by MS/MS. The gel was cut into ten slices, separating bands with abundant proteins from those with lower protein content. (d) Systematic identification of meiotic chromatin-associated proteins (MCAPs) by subtractive analysis of three proteomic data sets. Proteins represented with at least three unique peptides in P18 testes, but absent from both P6 and XXY*testes, were considered candidate meiotic chromatin-associated proteins. (e) Association of MEIOB with chromatin in P18 testes. Western blot analysis was performed using 20 μg protein from cytoplasmic extract, nuclear extract and chromatin. TEX19 and histone H3 serve as cytoplasmic and chromatin controls, respectively. (f) MEIOB protein expression in adult mouse tissues. ACTB serves as a loading control. Note that heart and skeletal muscle contain little ACTB. Protein molecular mass standards are shown in kDa. Figure 1: Proteomic identification of meiotic chromatin-associated proteins from mouse testes. ( a ) Biochemical purification of chromatin from P18 testes. ( b ) Purity assessment of isolated meiotic chromatin by western blotting. SYCP2 is known to associate with meiotic chromatin. TEX19 is a cytoplasmic protein control. Histone H3 is a ubiquitous chromatin-associated protein. ( c ) Identification of chromatin-associated proteins by MS/MS. The gel was cut into ten slices, separating bands with abundant proteins from those with lower protein content. ( d ) Systematic identification of meiotic chromatin-associated proteins (MCAPs) by subtractive analysis of three proteomic data sets. Proteins represented with at least three unique peptides in P18 testes, but absent from both P6 and XX Y* testes, were considered candidate meiotic chromatin-associated proteins. ( e ) Association of MEIOB with chromatin in P18 testes. Western blot analysis was performed using 20 μg protein from cytoplasmic extract, nuclear extract and chromatin. TEX19 and histone H3 serve as cytoplasmic and chromatin controls, respectively. ( f ) MEIOB protein expression in adult mouse tissues. ACTB serves as a loading control. Note that heart and skeletal muscle contain little ACTB. Protein molecular mass standards are shown in kDa. Full size image In addition to meiotic cells, P18 testes contain mitotic germ cells and somatic cells ( Fig. 1d ). To identify proteins only associated with meiotic chromatin, we applied a subtractive approach, excluding chromatin-associated proteins present in mitotic cells. Using the same biochemical/proteomics protocol, we identified chromatin-associated proteins from postnatal day 6 (P6) mouse testes, which contain spermatogonia but no meiotic cells [14] , and from XX Y* testes, which lack all germ cells and thus contain only somatic cells [15] . By subtracting these two data sets from the P18 data set, with a stringent cutoff value of at least 3 unique peptides in P18 but none in P6 and XX Y* , we identified 51 putative meiotic chromatin-associated proteins ( Fig. 1d and Supplementary Table S1 ). Identification of previously known meiotic chromatin-associated proteins confirmed the validity of our approach: 13 of 51 proteins identified are known to localize to meiotic chromatin (SYCP1, SYCP2, SYCP3, SYCE2, SMC1B, HORMAD1, H2AX, MDC1, TERF1, TDP1, PIWIL1, PIWIL2 and YBX2; Supplementary Table S1 ), including all three synaptonemal complex proteins. Furthermore, the genes encoding 19 proteins identified in our screen had been subjected to targeted deletion in mice: 11 mutants exhibited meiotic arrest, 2 showed post-meiotic spermiogenic arrest, 4 displayed embryonic lethality (with an unknown role in meiosis) and 2 were dispensable for fertility. The identification of these known meiosis factors validates our biochemical/proteomic approach and suggests that the other 32 proteins identified in our screen are likely to be novel meiotic chromatin-associated proteins ( Supplementary Table S1 ). MEIOB is a novel meiosis-specific protein To test whether the newly identified putative meiotic chromatin-associated proteins indeed localize to meiotic chromatin and function in meiosis, we focused on one of these uncharacterized proteins—MEIOB. MEIOB (470 amino acids (aa)) is predicted to contain an OB fold (aa 167–272) with limited homology to the ssDNA-binding domain-B OB domain of RPA1 ( Supplementary Fig. S1 ). MEIOB homologues are present in mammals, chicken, fugu fish, Drosophila and Arabidopsis . Western blot analyses using specific antibodies raised against MEIOB confirmed its association with chromatin; MEIOB was also detectable in the cytoplasmic and soluble nuclear fractions of the testis ( Fig. 1e ). Although abundantly expressed in the testis, MEIOB was not detectable in somatic tissues when examined by western blotting ( Fig. 1f ). MEIOB localized predominantly to the nuclei of spermatocytes in the testis ( Supplementary Fig. S2 ). Therefore, MEIOB is a novel meiotic chromatin-associated protein. MEIOB co-localizes with RPA in foci on meiotic chromosomes Immunostaining of spread nuclei of spermatocytes showed that MEIOB formed discrete foci on chromosomes, foci that exhibited a dynamic distribution pattern during meiosis ( Fig. 2a–j ). MEIOB foci were absent at the early leptotene stage ( Fig. 2a ), became first detectable on late leptotene chromosomes ( Fig. 2b ), formed arrays along synaptonemal complexes in zygotene and early pachytene spermatocytes ( Fig. 2c,d ), and disappeared in late pachytene spermatocytes ( Fig. 2e ). At a range of 100–200 per cell, MEIOB foci peaked at the zygotene stage ( Fig. 2k ). Notably, MEIOB foci were formed along the partially synapsed sex chromosomes at the pachytene stage ( Fig. 2d ). In addition, MEIOB formed foci on meiotic chromosomes in fetal oocytes ( Supplementary Fig. S3 ), implying functional relevance of MEIOB for meiosis in both sexes. MEIOB was absent from the adult ovary ( Fig. 1f ), in which oocytes are at the diplotene stage. No focal staining was observed in Meiob −/− spermatocytes with the antibody used for these analyses, demonstrating that the antibody is specific for MEIOB and does not crossreact with RPA1 ( Supplementary Fig. S4a ). 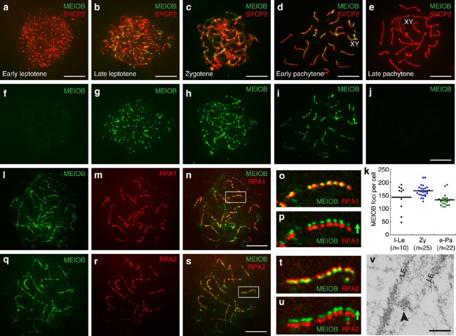Figure 2: MEIOB co-localizes with RPA in foci on meiotic chromosomes. (a–e) Distribution pattern of MEIOB foci on chromatin of spermatocytes from early leptotene through late pachytene stages. (f,j) the same cells ina–eare shown with MEIOB labelling only. (k) Number of MEIOB foci in spermatocytes at successive stages of meiotic prophase I. Stages were determined by SYCP2 staining. l-Le, late leptotene; Zy, zygotene; e-Pa, early pachytene;n, number of cells counted. The line indicates the average. (l–p) MEIOB co-localizes with RPA1 on the meiotic chromosomes of spermatocytes. The same spermatocyte is shown with MEIOB labelling only (l), RPA1 labelling only (m) and in a merged image (n). Enlarged views of the marked chromosome innare shown inoandp(without or with offset channels). (q–u) MEIOB co-localizes with RPA2 on the meiotic chromosomes of spermatocytes. The same spermatocyte is shown with MEIOB labelling only (q), RPA2 labelling only (r) and in a merged image (s). Enlarged views of the marked chromosome insare shown intandu(without or with offset channels). (v) Electron microscopy with immunogold (6 nm particles, arrowhead)-labelled MEIOB reveals signal between the lateral elements (LE) in spermatocytes. Scale bars, 10 μm (a–s); 0.2 μm (v). Figure 2: MEIOB co-localizes with RPA in foci on meiotic chromosomes. ( a – e ) Distribution pattern of MEIOB foci on chromatin of spermatocytes from early leptotene through late pachytene stages. ( f , j ) the same cells in a – e are shown with MEIOB labelling only. ( k ) Number of MEIOB foci in spermatocytes at successive stages of meiotic prophase I. Stages were determined by SYCP2 staining. l-Le, late leptotene; Zy, zygotene; e-Pa, early pachytene; n , number of cells counted. The line indicates the average. ( l – p ) MEIOB co-localizes with RPA1 on the meiotic chromosomes of spermatocytes. The same spermatocyte is shown with MEIOB labelling only ( l ), RPA1 labelling only ( m ) and in a merged image ( n ). Enlarged views of the marked chromosome in n are shown in o and p (without or with offset channels). ( q – u ) MEIOB co-localizes with RPA2 on the meiotic chromosomes of spermatocytes. The same spermatocyte is shown with MEIOB labelling only ( q ), RPA2 labelling only ( r ) and in a merged image ( s ). Enlarged views of the marked chromosome in s are shown in t and u (without or with offset channels). ( v ) Electron microscopy with immunogold (6 nm particles, arrowhead)-labelled MEIOB reveals signal between the lateral elements (LE) in spermatocytes. Scale bars, 10 μm ( a – s ); 0.2 μm ( v ). Full size image We next evaluated the potential interaction of MEIOB with other meiotic recombination-related proteins and found that MEIOB co-localized with RPA, which forms foci on prophase I meiotic chromosomes [16] , [17] , [18] . Immunofluorescence analyses with antibodies specific for both the RPA1 and RPA2 subunits of RPA confirmed complete focal association with MEIOB ( Fig. 2l–u ). As previously shown, RPA foci gradually replace RAD51 foci during meiotic recombination; thus, only a subset of RPA foci overlap with RAD51 foci [17] . The relative distribution pattern of MEIOB and RAD51 foci is similar to that of RPA and RAD51 foci. Early leptotene spermatocytes contained a large number of RAD51 foci but lacked MEIOB foci ( Supplementary Fig. S5a ). In zygotene and pachytene spermatocytes ( Supplementary Fig. S5b–g ), the distribution of MEIOB and RAD51 foci appeared to be dynamic: some foci contained both proteins, some contained RAD51 only and others contained MEIOB only. RAD51 and DMC1 always co-localize in foci on meiotic chromosomes [19] . As expected, MEIOB co-localized with DMC1 in only a subset of foci ( Supplementary Fig. S6a–d′ ). In a subset of foci, MEIOB also co-localized with MSH4, a member of the ZMM group involved in meiotic recombination ( Supplementary Fig. S6e–h′ ) [20] . Thus, MEIOB and RPA always co-localize, whereas MEIOB co-localizes with RAD51, DMC1 or MSH4 only in a subset of foci. Ultrastructural analysis by immunogold electron microscopy showed MEIOB signal in the electron-dense nodule between lateral elements of the synaptonemal complex ( Fig. 2v ). These results suggest that MEIOB associates with RPA during meiotic recombination. MEIOB binds to ssDNA A central OB domain is the only predicted protein motif in MEIOB ( Fig. 3a ). OB folds are compact barrel-like structures that can recognize and interact with single-stranded nucleic acids or those with an unusual structure [21] , [22] . We expressed the central region of MEIOB including the OB fold (aa 136–307; Fig. 3a , construct A) as a glutathione S -transferase (GST) fusion protein and assessed its nucleic acid binding capacity. Truncated MEIOB (construct A) bound to ssDNA with an apparent K d of 0.4 μ M ( Fig. 3b,c ). Truncated MEIOB exhibited high affinity for ssDNA at least 24 nucleotides (nt) in length and lower affinity for shorter fragments ( Fig. 3d ). Truncated MEIOB also bound to dsDNA with 5′- or 3′-single-stranded flaps, but not to dsDNA with blunt ends ( Fig. 3e ). These experiments demonstrate that MEIOB is an ssDNA-binding protein. 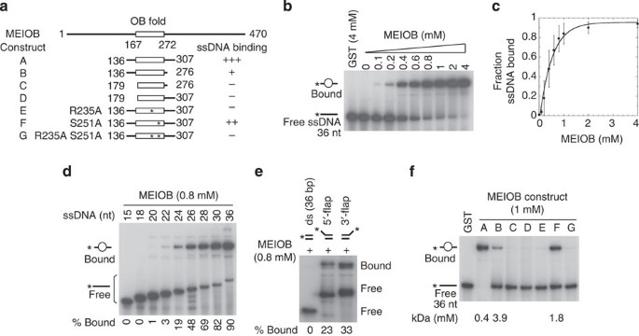Figure 3: MEIOB binds to ssDNA but not dsDNA. (a) MEIOB contains an OB fold. All MEIOB constructs were expressed as GST fusion proteins. Only construct A (MEIOB central region; aa 136–307) was used in experiments illustrated inbthroughe. The summary of ssDNA-binding activity is based on the results from panelf: +++, strong; ++, intermediate; +, weak; −, no binding. TheKdvalues are shown inf. (b) Truncated MEIOB binds to ssDNA. The ssDNA (d36GT) was 5′-labelled with32P (indicated by asterisk). (c) Binding curve for truncated MEIOB-ssDNA (d36GT) from triplicate electrophoretic mobility shift assay (EMSA) experiments (mean±s.d.). (d) Binding of truncated MEIOB to ssDNA oligonucleotides of various lengths. All oligonucleotides [d(GT)nor d(GT)nG] were 5′-32P-labelled. (e) Truncated MEIOB binds to 5′- and 3′-ssDNA flap (30 nt) but not dsDNA. One strand of the dsDNA and the 5′-flap DNA were 5′-32P-labelled. The long strand in the 3′-flap DNA was 3′-32P-labelled. (f) EMSA analysis of various MEIOB constructs depicted ina. GST was used as negative control. Figure 3: MEIOB binds to ssDNA but not dsDNA. ( a ) MEIOB contains an OB fold. All MEIOB constructs were expressed as GST fusion proteins. Only construct A (MEIOB central region; aa 136–307) was used in experiments illustrated in b through e . The summary of ssDNA-binding activity is based on the results from panel f : +++, strong; ++, intermediate; +, weak; −, no binding. The K d values are shown in f . ( b ) Truncated MEIOB binds to ssDNA. The ssDNA (d36GT) was 5′-labelled with 32 P (indicated by asterisk). ( c ) Binding curve for truncated MEIOB-ssDNA (d36GT) from triplicate electrophoretic mobility shift assay (EMSA) experiments (mean±s.d.). ( d ) Binding of truncated MEIOB to ssDNA oligonucleotides of various lengths. All oligonucleotides [d(GT) n or d(GT) n G] were 5′- 32 P-labelled. ( e ) Truncated MEIOB binds to 5′- and 3′-ssDNA flap (30 nt) but not dsDNA. One strand of the dsDNA and the 5′-flap DNA were 5′- 32 P-labelled. The long strand in the 3′-flap DNA was 3′- 32 P-labelled. ( f ) EMSA analysis of various MEIOB constructs depicted in a . GST was used as negative control. Full size image To identify essential elements of the ssDNA-binding domain of MEIOB, we expressed protein segments with additional amino- and carboxy-terminal truncations and point mutations (constructs B–G; Fig. 3a,f ). We found that deletion of aa 277–307, located C-terminal to the OB fold, resulted in a tenfold reduction in the binding affinity ( K d for construct B: 3.9 μ M ), whereas deletion of aa 136–178 (construct C) abolished DNA-binding activity. On the basis of the crystal structure of human RPA1 ( [23] ), several residues in the ssDNA-binding domain-B OB domain are involved in DNA binding; these are conserved in the MEIOB OB domain ( Supplementary Fig. S1 ). Analysis of mutant protein segments with point mutations at such residues identified R235 of MEIOB to be essential for DNA binding. Residue S251 was important but not required for DNA binding, as the S251A mutation reduced the binding affinity by 4.5-fold ( K d for construct F: 1.8 μ M ). MEIOB exhibits ssDNA-specific 3′–5′ exonuclease activity When the in vitro binding assays with 5′- 32 P-labelled ssDNA were performed in the presence of Mg 2+ , a cleaved product appeared proportionally to MEIOB concentration, revealing that truncated MEIOB (construct A in Fig. 3a ) exhibits Mg 2+ -dependent nuclease activity ( Fig. 4a ). Truncated MEIOB cleaved ssDNA into oligonucleotides of six to predominantly eight bases in length ( Fig. 4b ). Although its binding affinity to oligonucleotides of ≤18 nt was low ( Fig. 3d ), truncated MEIOB cleaved ssDNA fragments as short as 10–15 nt into 8-nt oligonucleotides ( Fig. 4c ). The generation of 5′-labelled 6- to 8-nt products indicated that truncated MEIOB has either endonuclease or 3′-exonuclease activity. Truncated MEIOB did not process 5′-flap ssDNA, showing that it lacks 5′-exonuclease or endonuclease activity ( Fig. 4d ). Rather, truncated MEIOB cleaved nucleotides from the 3′-end of 3′-radiolabelled oligos ( Fig. 4e ), demonstrating that it is a 3′-exonuclease. The 3′-exonuclease activity of truncated MEIOB was robust for ssDNA of ≥18 nt and lower for shorter oligonucleotides (5–15 nt; Fig. 4e ), suggesting that the enzymatic activity of truncated MEIOB increases with stronger DNA binding. The ability of truncated MEIOB to digest the 3′-flap DNA further validated its 3′-exonuclease activity ( Fig. 4f ). The exonuclease activity of truncated MEIOB on the 3′-flap was similar to that on ssDNA. Truncated MEIOB digested 3′-flaps efficiently to ~8 nt, digested 6- and 8-nt 3′-flaps very inefficiently, but had no effect on 4-nt 3′-flaps ( Fig. 4g ). At 0.8 μ M , truncated MEIOB digested ssDNA efficiently only to a length of 8 nt after 10 min of incubation ( Fig. 4h ). With a tenfold excess (8 μ M ), truncated MEIOB further digested ssDNA to <5 nt or even completely ( Fig. 4h ). In conclusion, truncated MEIOB exhibits 3′-exonuclease activity specific for ssDNA in vitro . However, we cannot exclude the possibility that in vitro biochemical analyses on truncated MEIOB proteins may not reflect precisely the activity of the full-length protein in vitro , in vivo , or in partner with other proteins. 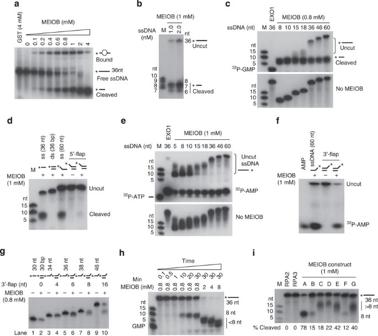Figure 4: MEIOB exhibits ssDNA-specific 3′-exonuclease activity. Construct A (MEIOB central region,Fig. 3a) (aa 136–307) was used in experiments illustrated inathroughh. (a) Truncated MEIOB exhibits nuclease activity in addition to its ssDNA-binding activity. (b) Size determination of 5′-labelled products generated by MEIOB. An 8-nt product was predominant. All products (bthroughi) were resolved on denaturing acrylamide gels. (c) Truncated MEIOB processes 5′-labelled oligonucleotides of various lengths.ExoI digests ssDNA completely. (d) Truncated MEIOB lacks nuclease activity on dsDNA and 5′-flap (30 nt) DNA substrates. (e) Truncated MEIOB exhibits 3′-exonuclease activity on 3′-labelled oligonucleotides of various lengths. EXO1 serves as a positive control. (f) Truncated MEIOB efficiently processes oligonucleotides with a 3′-flap (30 nt). (g) Extent of 3′-flap digestion by truncated MEIOB. (h) Time-course and gradient analyses of truncated MEIOB nuclease activity. Note that MEIOB at higher concentrations (2 to 8 μM) produced shorter end products (<8 nt). (i) Nuclease activities of various MEIOB mutants shown inFig. 3a. Recombinant GST-RPA2 and -RPA3 were used as negative controls. Per cent (%) cleavage represents the average from three independent experiments. Figure 4: MEIOB exhibits ssDNA-specific 3′-exonuclease activity. Construct A (MEIOB central region, Fig. 3a ) (aa 136–307) was used in experiments illustrated in a through h . ( a ) Truncated MEIOB exhibits nuclease activity in addition to its ssDNA-binding activity. ( b ) Size determination of 5′-labelled products generated by MEIOB. An 8-nt product was predominant. All products ( b through i ) were resolved on denaturing acrylamide gels. ( c ) Truncated MEIOB processes 5′-labelled oligonucleotides of various lengths. Exo I digests ssDNA completely. ( d ) Truncated MEIOB lacks nuclease activity on dsDNA and 5′-flap (30 nt) DNA substrates. ( e ) Truncated MEIOB exhibits 3′-exonuclease activity on 3′-labelled oligonucleotides of various lengths. EXO1 serves as a positive control. ( f ) Truncated MEIOB efficiently processes oligonucleotides with a 3′-flap (30 nt). ( g ) Extent of 3′-flap digestion by truncated MEIOB. ( h ) Time-course and gradient analyses of truncated MEIOB nuclease activity. Note that MEIOB at higher concentrations (2 to 8 μM) produced shorter end products (<8 nt). ( i ) Nuclease activities of various MEIOB mutants shown in Fig. 3a . Recombinant GST-RPA2 and -RPA3 were used as negative controls. Per cent (%) cleavage represents the average from three independent experiments. Full size image We next tested the nuclease activity of various MEIOB mutants with truncations and point mutations ( Fig. 3a ). We found that all the mutant proteins exhibited much lower nuclease activities than construct A ( Fig. 4i ). Interestingly, similar to construct A, constructs B and F digested the 36 nt ssDNA to 8 nt. In contrast, constructs C, D, E and G produced digested oligonucleotides longer than 8 nt, suggesting lower enzymatic processivity. As constructs A, B and F bind to ssDNA, but C, D, E and G do not ( Fig. 3f ), these data suggest that the DNA-binding property of MEIOB might stimulate its enzymatic processivity. MEIOB is required for meiosis and fertility in both sexes To uncover the requirement of MEIOB for meiosis, we disrupted the Meiob gene ( Fig. 5a ). Meiob −/− mice were viable and appeared to be healthy. Western blotting demonstrated the absence of MEIOB protein in Meiob −/− testes ( Fig. 5b ), confirming that the Meiob mutant was null. Interbreeding of heterozygous ( Meiob +/− ) mice yielded a normal Mendelian ratio (182:357:169) of Meiob +/+ , Meiob +/− , and Meiob −/− offspring. 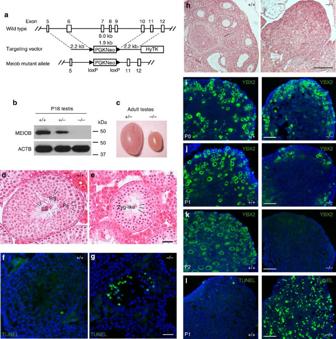Figure 5: MEIOB is required for meiosis and fertility in mice of both sexes. (a) Targeted inactivation of theMeiobgene. The mouseMeiobgene maps to chromosome 17 and has 14 exons. Deletion of exons 6–10 (aa 111–293) is expected to cause a frame shift in the resulting transcript. (b) Absence of MEIOB protein in P18Meiob−/−testis. (c) Significant size reduction in 8-week-oldMeiob−/−testis. (d,e) Histological analysis of 8-week-old wild-type andMeiob−/−testes. Zyg, zygotene spermatocytes; Pa, pachytene spermatocytes; RS, round spermatids; ES, elongated spermatids. (f,g) TUNEL analysis of wild-type andMeiob−/−seminiferous tubules. Note the large number of apoptotic cells (green) inMeiob−/−tubules. Scale bar, 25 μm (e,g). (h) Histological analysis of ovaries from adult wild-type andMeiob−/−mice. Scale bar, 50 μm. (i–k) Progressive loss of oocytes inMeiob−/−ovaries. Frozen sections prepared from postnatal day P0, P1 and P2 wild-type andMeiob−/−ovaries were immunolabelled with anti-YBX2 antibodies. (l) TUNEL analysis of P1 ovaries. Nuclear DNA (i–l) was counterstained with 4',6-diamidino-2-phenylindole (DAPI; blue). Scale bars, 50 μm (i–l). Figure 5: MEIOB is required for meiosis and fertility in mice of both sexes. ( a ) Targeted inactivation of the Meiob gene. The mouse Meiob gene maps to chromosome 17 and has 14 exons. Deletion of exons 6–10 (aa 111–293) is expected to cause a frame shift in the resulting transcript. ( b ) Absence of MEIOB protein in P18 Meiob −/− testis. ( c ) Significant size reduction in 8-week-old Meiob −/− testis. ( d , e ) Histological analysis of 8-week-old wild-type and Meiob −/− testes. Zyg, zygotene spermatocytes; Pa, pachytene spermatocytes; RS, round spermatids; ES, elongated spermatids. ( f , g ) TUNEL analysis of wild-type and Meiob −/− seminiferous tubules. Note the large number of apoptotic cells (green) in Meiob −/− tubules. Scale bar, 25 μm ( e , g ). ( h ) Histological analysis of ovaries from adult wild-type and Meiob −/− mice. Scale bar, 50 μm. ( i – k ) Progressive loss of oocytes in Meiob −/− ovaries. Frozen sections prepared from postnatal day P0, P1 and P2 wild-type and Meiob −/− ovaries were immunolabelled with anti-YBX2 antibodies. ( l ) TUNEL analysis of P1 ovaries. Nuclear DNA ( i – l ) was counterstained with 4',6-diamidino-2-phenylindole (DAPI; blue). Scale bars, 50 μm ( i – l ). Full size image Both Meiob −/− males and females were sterile. Disruption of Meiob resulted in dramatically reduced testis size ( Fig. 5c ). Testes from 8-week-old Meiob −/− males weighed 70% less than wild type (54.5±6.7 mg versus 184.0±10.5 mg per pair; n =4; Student’s t -test, P <0.0001). Histological analysis revealed complete meiotic arrest in germ cells of Meiob −/− adult males ( Fig. 5d,e ). In contrast to wild-type seminiferous tubules that contained a full spectrum of germ cells ( Fig. 5d ), tubules from Meiob −/− testes completely lacked post-meiotic germ cells, with zygotene-like spermatocytes reflecting the most advanced germ cells ( Fig. 5e ). In addition, 3-week-old Meiob −/− testis also exhibited a block in meiosis, showing that inaction of Meiob causes meiotic failure during the first wave of spermatogenesis and in adults ( Supplementary Fig. S7 ). TdT-mediated dUTP nick end labeling (TUNEL) assays showed that Meiob -deficient spermatocytes underwent apoptosis ( Fig. 5g ), suggesting that mutant spermatocytes are eliminated at the pachytene checkpoint [24] . Ovaries from adult Meiob −/− female mice were small and devoid of oocytes of any developmental stage ( Fig. 5h ). To determine the time point of oocyte loss, we examined ovaries at different ages, using anti-YBX2 antibodies to identify oocytes [25] . Meiob −/− ovaries contained an abundant number of oocytes at birth (P0, Fig. 5i ), but were almost devoid of oocytes by postnatal day 1 ( Fig. 5j ), with complete lack of oocytes by day 2 ( Fig. 5k ). TUNEL assays revealed that oocytes in Meiob −/− ovaries underwent massive apoptosis at postnatal day 1 ( Fig. 5l ), which is in agreement with a complete oocyte loss within the first 2 days after birth. Complete early postnatal loss of oocytes is characteristic of recombination-defective ( Dmc1 , Msh5 or Atm ) mouse mutants [26] . Therefore, MEIOB is essential for meiosis in both sexes. MEIOB is required for chromosomal synapsis To elucidate the molecular defects of Meiob -deficient meiotic germ cells, we monitored the process of chromosomal synapsis by assessing the distribution of proteins of the central (SYCP1) and axial/lateral elements (SYCP2) of synaptonemal complexes ( Supplementary Fig. S8 ) [12] , [27] . In leptotene spermatocytes, the axial elements marked by SYCP2 began to form but SYCP1 filaments were not yet detectable ( Supplementary Fig. S8a ). At the zygotene stage, axial elements are normally fully formed and chromosomes progressively synapse. However, Meiob −/− spermatocytes exhibited severe defects in chromosomal synapsis ( Supplementary Fig. S8b–h ): 40% of Meiob −/− spermatocytes formed long axial elements, suggesting progression to the zygotene stage; however, these cells completely lacked synapsis ( Supplementary Fig. S8b ). Such cells were not observed in wild-type males ( Supplementary Fig. S8h ). In wild-type postnatal day 16 testes, ~65% of spermatocytes reached the pachytene stage. No normal pachytene spermatocytes were observed in Meiob −/− males ( Supplementary Fig. S8h ), but ~15% of Meiob −/− spermatocytes appeared to be at a pachytene-like stage, with shortened axial elements, suggesting chromosomal condensation, but no evidence for synapsis ( Supplementary Fig. S8f, h ). These results demonstrate that MEIOB is essential for chromosomal synapsis. Meiob −/− mice exhibit defects in meiotic recombination We next examined the process of meiotic recombination. During meiosis, SPO11-generated DSBs lead to phosphorylation of H2AX through the activation of the ataxia telangiectasia mutated kinase [28] , [29] , [30] . Ataxia telangiectasia and Rad3-related protein (ATR) is recruited to unsynapsed chromosomes and phosphorylates H2AX at the zygotene and pachytene stages [31] , [32] . Recombinases RAD51/DMC1 together with the HOP2-MND1 heterodimer direct strand invasion into the homologous chromosomes, resulting in D-loop formation [33] . RPA may bind to the D-loop, whereas ZMM proteins such as MSH4 and TEX11 facilitate the formation of crossovers [20] , [34] . These proteins form recombination nodules and can be visualized as foci on meiotic chromosomes [35] . Analysis of chromosome spreads from Meiob −/− spermatocytes revealed the presence of the majority of recombination factors assessed: γH2AX persisted on chromatin and ATR formed foci on synaptonemal complexes ( Supplementary Fig. S9 ). These results are in agreement with the severe synaptic defects in Meiob −/− spermatocytes ( Supplementary Fig. S8 ). The initial numbers of RAD51 and DMC1 foci between wild-type and Meiob −/− spermatocytes were similar at leptotene ( Fig. 6a,b ). The numbers of RAD51, DMC1, RPA and TEX11 foci were also comparable between wild-type and Meiob −/− spermatocytes at the zygotene stage ( Fig. 6a–d ). Interestingly, in the Meiob −/− pachytene-like spermatocytes, the number of RAD51 and DMC1 foci decreased as expected, but RPA foci persisted ( Fig. 6c ), suggesting that in the absence of MEIOB, meiotic recombination fails after strand invasion, or RAD51/DMC1 filament is unstable and falls off, leading to replacement by RPA1. 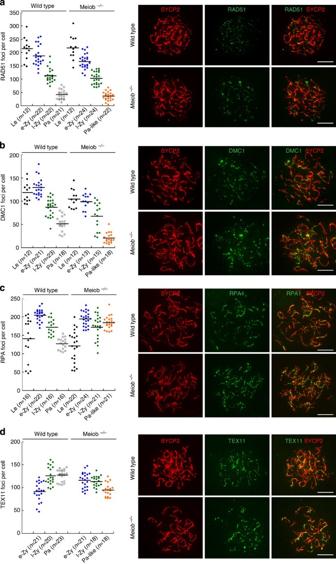Figure 6: MEIOB is essential for meiotic recombination. Immunolabelling for proteins of the synaptonemal complex (SYCP2, lateral elements) and recombination nodules was performed on spread nuclei of spermatocytes from wild-type andMeiob−/−testes at postnatal day 16. The meiotic stages of spermatocytes were determined based on the morphology of the synaptonemal complexes. Spermatocytes were categorized into the following groups: leptotene (Le), early-mid zygotene (e-Zy), late zygotene (l-Zy) and pachytene (Pa). Pachytene-like (Pa-like) spermatocytes contained prominent but short lateral elements (seeSupplementary Fig. S8f). Pa-like spermatocytes were present inMeiob−/−testes but absent in wild-type testes. Dot plots for each DNA repair protein show the number of foci per cell; solid lines designate the average for each spermatocyte category;n, number of cells counted. Representative images of spermatocytes at early-mid zygotene stages are shown in separate channels and as merged images. (a) RAD51 foci. (b) DMC1 foci. (c) RPA foci. (d) TEX11 foci. Scale bars, 10 μm. Figure 6: MEIOB is essential for meiotic recombination. Immunolabelling for proteins of the synaptonemal complex (SYCP2, lateral elements) and recombination nodules was performed on spread nuclei of spermatocytes from wild-type and Meiob −/− testes at postnatal day 16. The meiotic stages of spermatocytes were determined based on the morphology of the synaptonemal complexes. Spermatocytes were categorized into the following groups: leptotene (Le), early-mid zygotene (e-Zy), late zygotene (l-Zy) and pachytene (Pa). Pachytene-like (Pa-like) spermatocytes contained prominent but short lateral elements (see Supplementary Fig. S8f ). Pa-like spermatocytes were present in Meiob −/− testes but absent in wild-type testes. Dot plots for each DNA repair protein show the number of foci per cell; solid lines designate the average for each spermatocyte category; n , number of cells counted. Representative images of spermatocytes at early-mid zygotene stages are shown in separate channels and as merged images. ( a ) RAD51 foci. ( b ) DMC1 foci. ( c ) RPA foci. ( d ) TEX11 foci. Scale bars, 10 μm. Full size image At the mid-late pachytene stage, MLH1 foci become apparent in normal spermatocytes, marking sites of crossover [36] , [37] . Meiob −/− spermatocytes did not progress to the mid-late pachytene stage and, thus, were devoid of MLH1 foci. The meiotic defects in fetal oocytes were similar to those observed in spermatocytes from Meiob −/− mice. However, a small percentage of Meiob −/− oocytes (7%) advanced to the pachytene stage with full synapsis by 17.5 days of embryonic development, whereas 93% of Meiob +/− oocytes developed to this stage. This difference with males may result from the possibility that Meiob −/− oocytes proceed in meiosis with some synapsis defects, which may be overcome with time, whereas mutant spermatocytes with synapsis defects are rapidly eliminated. All Meiob −/− pachytene oocytes ( n =30) were γH2AX-positive, indicating that DSBs were not repaired and lacked MLH1 foci ( Supplementary Fig. S10 ). Our results demonstrate that the markers of early steps of meiotic recombination (DSB formation, 5′-end resection and strand invasion) are present in the absence of MEIOB, but that markers of subsequent steps of meiotic recombination are lacking. Our results suggest that defective chromosomal synapsis in Meiob −/− mice is likely to be attributed to defects in meiotic recombination. MEIOB forms complexes with RPA2 and SPATA22 To identify protein partners of MEIOB, we performed immunoprecipitation (IP) with testicular extracts using anti-MEIOB antibodies and identified a single prominent band that was present in the immunoprecipitated proteins from wild-type but absent from Meiob −/− testes ( Fig. 7a ). MS/MS analysis revealed that this band contained RPA2 and SPATA22, a meiosis-specific protein [38] . To verify the association of MEIOB with RPA2 and SPATA22, we performed co-IP experiments followed by western blot analysis and confirmed that RPA2 and SPATA22 were present in the protein fraction immunoprecipitated with the anti-MEIOB antibody ( Fig. 7b ). We found that SPATA22, similar to MEIOB, formed discrete foci on meiotic chromosomes ( Fig. 7c and Supplementary Fig. S4b ). Specificity of the SPATA22 antibody was confirmed by the absence of foci in Spata22 −/− spermatocytes ( Supplementary Fig. S4b ). In addition, SPATA22 co-localized with MEIOB in foci on meiotic chromosomes from spermatocytes ( Supplementary Fig. S11 ). These studies demonstrate that MEIOB forms protein complexes with RPA and with SPATA22 in the testis. 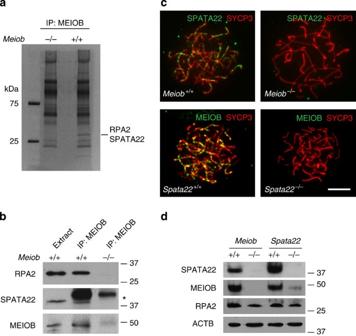Figure 7: MEIOB forms complexes with RPA2 and SPATA22. (a) Identification of MEIOB-associated proteins from P18 testes by IP and mass spectrometry. The gel was stained with SYPRO Ruby. (b) Co-IP analysis of MEIOB with RPA2 and SPATA22 from testicular protein extracts. The asterisk indicates a nonspecific band. (c) Interdependent localization of MEIOB and SPATA22 on meiotic chromosomes from spermatocytes.Spata22−/−refers toSpata22repro42/repro42mice38. Scale bar, 10 μm. (d) Western blot analysis of MEIOB and SPATA22 proteins in testes from wild-type,Meiob−/−andSpata22−/−mutant mice. Figure 7: MEIOB forms complexes with RPA2 and SPATA22. ( a ) Identification of MEIOB-associated proteins from P18 testes by IP and mass spectrometry. The gel was stained with SYPRO Ruby. ( b ) Co-IP analysis of MEIOB with RPA2 and SPATA22 from testicular protein extracts. The asterisk indicates a nonspecific band. ( c ) Interdependent localization of MEIOB and SPATA22 on meiotic chromosomes from spermatocytes. Spata22 −/− refers to Spata22 repro42/repro42 mice [38] . Scale bar, 10 μm. ( d ) Western blot analysis of MEIOB and SPATA22 proteins in testes from wild-type, Meiob −/− and Spata22 −/− mutant mice. Full size image Interdependent localization of MEIOB and SPATA22 RPA foci were formed on Meiob -null meiotic chromosomes ( Fig. 6c ), indicating that the interaction of RPA with meiotic chromatin is independent of MEIOB. In stark contrast, SPATA22 foci were absent in Meiob -null spermatocytes and MEIOB foci were absent in Spata22 -null spermatocytes ( Fig. 7c ), suggesting that MEIOB and SPATA22 can interact with meiotic chromosomes only in the presence of each other. Reciprocal interdependence between these two proteins was further supported by the observation that SPATA22 protein was absent in Meiob −/− testes and MEIOB protein was nearly absent in Spata22 −/− testes ( Fig. 7d ). These results also indicate that the stability of these two proteins depends on their coexpression and interaction. Consistent with this hypothesis, the Meiob mutant phenocopies the meiotic failure observed in Spata22 -null male and female mice [38] . SPATA22 has no recognizable domains, whereas MEIOB binds to ssDNA and exhibits 3′-exonuclease activity. These results suggest that MEIOB may function as the catalytic subunit of this novel meiotic recombination complex that requires SPATA22 as an essential cofactor. Genetic and cytological studies in diverse organisms from yeast to humans have yielded a wealth of knowledge on meiosis. However, more than in other model organisms, approaches to gain insight into mammalian meiosis have been hampered by various obstacles. Here we have developed a biochemical and proteomics strategy to systematically identify meiotic chromatin-associated proteins. Our strategy has been proven to be highly successful, identifying synaptonemal complex components, proteins critical for meiotic recombination and factors involved in chromatin modification. In this report, we have characterized the essential function of one novel meiotic chromatin-associated protein—MEIOB. Furthermore, these proteomic screen and functional studies set the stage for future characterization of other novel putative meiotic chromatin-associated proteins ( Supplementary Table S1 ). Many key steps of meiotic recombination, such as second-end capture, are poorly understood. Biochemical and genetic studies have shown that yeast RAD52 has a key role in second-end capture [39] , [40] , [41] , [42] . In biochemical assays, mammalian RAD52 also mediates second-end capture [43] . However, RAD52-deficient mice display no abnormalities in viability and fertility, suggesting that RAD52 is not essential for recombination in mice, and that other genes may functionally substitute RAD52 in mice [44] . Our results support a model in which MEIOB and its cofactor SPATA22 may mediate second-end capture during mammalian meiotic recombination ( Fig. 8 ). MEIOB is not required for the early steps of meiotic recombination, including DSB formation, end resection and strand invasion. However, crossovers are never formed in Meiob -deficient germ cells and, in normal pachytene spermatocytes, the disappearance of MEIOB foci precedes the appearance of crossovers. These results indicate that MEIOB is likely to function at the time point after strand invasion ( Fig. 8 ). Similar to RAD52, MEIOB binds to ssDNA and interacts with RPA. Therefore, in our model, we propose that MEIOB mediates second-end capture through interactions with the RPA proteins, which coat both the D-loop and the resected second end. Second-end capture is a prerequisite to the double Holliday junction pathway ( Fig. 8 ) [45] . The severe synaptic defects and persistence of γH2AX caused by loss of MEIOB suggest that MEIOB is globally required for DSB repair during meiosis. 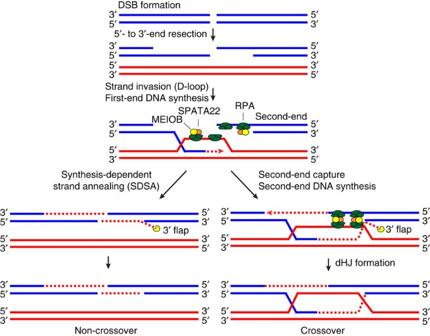Figure 8: Proposed model for MEIOB function during meiotic recombination. Key steps of meiotic recombination are illustrated. We propose that the RPA–MEIOB–SPATA22 complex coats both the D-loop and the ssDNA of the second end. In this model, the interaction between RPA and MEIOB–SPATA22 mediates second-end capture. Most DSBs are repaired through the synthesis-dependent strand annealing (SDSA) pathway, in which the D-loop collapses back to its sister chromatid. After the second-end capture, intermediates continue to form double Holliday junctions (dHJs), which are resolved into either crossovers or non-crossovers. We propose that MEIOB removes the 3′-flaps resulting from the first-end DNA synthesis in both dHJ and SDSA pathways. Figure 8: Proposed model for MEIOB function during meiotic recombination. Key steps of meiotic recombination are illustrated. We propose that the RPA–MEIOB–SPATA22 complex coats both the D-loop and the ssDNA of the second end. In this model, the interaction between RPA and MEIOB–SPATA22 mediates second-end capture. Most DSBs are repaired through the synthesis-dependent strand annealing (SDSA) pathway, in which the D-loop collapses back to its sister chromatid. After the second-end capture, intermediates continue to form double Holliday junctions (dHJs), which are resolved into either crossovers or non-crossovers. We propose that MEIOB removes the 3′-flaps resulting from the first-end DNA synthesis in both dHJ and SDSA pathways. Full size image We postulate that MEIOB may digest the 3′-ssDNA flap from the first end after annealing of the second end. After strand invasion, the first end primes DNA synthesis to extend the D-loop towards the second end. Subsequent to the second-end capture, the first end needs to be ligated to the resected strand of the second end. The first end-primed DNA synthesis could progress beyond the end point of the resected strand of the second end, such that a 3′-ssDNA flap forms after annealing of the D-loop with the single-stranded second end or after synthesis-dependent strand annealing ( Fig. 8 ). The timing of DSB end resection and first end-primed DNA synthesis is different; thus, generation of a gap or 3′-flap is expected after the second-end annealing. Whereas a gap can be filled by DNA synthesis, the repair of a 3′-flap requires different mechanisms. MEIOB may bind to and remove the 3′-flap through its nuclease activity, such that the ends can be ligated seamlessly without insertions. If 3′-flap is not processed, DNA helicases may act on this intermediate and destabilize it. In vivo , RPA may inhibit MEIOB activity on 3′-ends of ssDNA, thereby blocking promiscuous degradation. It is also possible that binding partners such as RPA and SPATA22 may modulate the nuclease activity and substrate specificity of MEIOB in vivo . In Drosophila and Arabidopsis , RPA1-related proteins (DmHDM and AtRPA1A) have evolved to regulate crossover formation, but neither is essential for meiotic recombination [46] , [47] . Although certain mitotic DNA repair proteins (such as RPA and RAD51) are utilized during meiotic recombination, many species have developed meiosis-specific repair machinery. One such factor is DMC1, a meiosis-specific paralogue of RAD51 (refs 48 , 49 , 50) . Yeast meiotic recombination only requires the D-loop forming activity of DMC1, whereas RAD51 has a supporting role [51] , [52] . DMC1 has evolved to initiate and engage the first interhomologue chromosome interaction unique to meiosis. Our results suggest that MEIOB might have evolved to drive another interhomologue interaction unique to meiosis—capture of the second homologue end. Biochemical purification of chromatin We optimized previously reported chromatin purification protocols ( Fig. 1a ) [10] , [11] as follows: 100 mg testis tissue was homogenized in 1 ml Buffer A (250 m M sucrose, 10 m M Tris-HCl, pH 8.0, 10 m M MgCl2, 1 m M EGTA, 1 × protease inhibitor cocktail III) and centrifuged at 300 g to separate nuclei (pellet) from cytoplasmic extract (supernatant). The nuclei were homogenized in Buffer B (Buffer A+0.1% Triton X-100, 0.25% NP-40) and centrifuged briefly at 100 g to remove nuclear membrane particles (pellet), which contain some chromatin (discarded). The chromatin-containing supernatant was layered over a 1.7 M sucrose cushion and centrifuged at 50,000 g for 1 h in an ultracentrifuge to remove soluble nuclear proteins and remnant cytoplasmic proteins/organelles. The pellet (chromatin) was washed three times, resuspended in Tris buffer, sonicated and boiled in an equal volume of 2 × SDS–PAGE buffer to dissolve all chromatin-associated proteins (~200 μg). Proteomics screen and mass spectrometry Seventy-five micrograms of chromatin-associated proteins from each testis sample were separated on a 10% SDS–PAGE gel ( Fig. 1c ) and stained with Coomassie blue. The gel lane was cut into ten slices, digested with trypsin and subjected to HPLC followed by MS/MS at the University of Pennsylvania Proteomic Core Facility. All spectra from ten MS/MS runs (one run/slice) were pooled and analysed using the Scaffold 2.6 software. A total of ~1,300 proteins were identified from each testis sample. Meiotic chromatin-associated proteins were identified by electronic subtraction using Scaffold 2.6 software as follows: meiotic chromatin-associated proteins=P18 testes−(P6 testes+XX Y* testes; Fig. 1d ). Recombinant proteins All recombinant GST fusion proteins were expressed in Escherichia coli (strain BL21) using the pGEX4T-1 vector. The complementary DNAs encoding mouse MEIOB, mouse RPA2 and mouse RPA3 were amplified by PCR from testis cDNAs and subcloned into the pGEX4T-1 vector. Point mutations in MEIOB were generated by PCR-based mutagenesis. All constructs were verified by sequencing. For induction, 3 ml of Luria broth (LB) medium (100 μg ml −1 ampicillin) was inoculated with a single colony, incubated for 6 h at 37 °C and used to inoculate 50 ml LB medium (100 μg ml −1 ampicillin) at 1:1,000 dilution. After overnight incubation, 50 ml culture was transferred to 600 ml fresh LB medium with ampicillin and continued to incubate at 37 °C till an absorbance at 600 nm of ~1.0. Isopropyl-β- D -thiogalactoside was added to a final concentration of 0.2 m M and the culture was incubated with shaking (180 r.p.m.) at 18 °C for 3 h. Bacteria were pelleted by centrifugation at 4 °C, resuspended in 20 ml cold DPBS buffer (Gibco 14190-136) and sonicated on ice. After centrifugation at 12,000 g for 20 min at 4 °C, the supernatant was transferred to a new tube. Three hundred microlitres of glutathione-Sepharose 4B beads (pretreated with cold PBS) was added to the lysate and incubated with continuous mixing for 2 h at 4 °C. The beads were pelleted by centrifugation for 1 min and washed nine times with 10 ml ice-cold PBS each. Proteins were eluted with 1 ml elution buffer (10 m M glutathione, 50 mM Tris-HCl, pH 8.0) for six times and the eluents were pooled. The eluted proteins were concentrated using the Pierce 20K MWCO concentrators (catalogue number 89886A, Thermo Scientific). Electrophoretic mobility shift and nuclease assays All biochemical assays were performed with purified recombinant GST-MEIOB proteins expressed in E. coli. Nuclease assays were performed for 30 min at room temperature with 1 μ M (or otherwise indicated) recombinant MEIOB protein and 2 n M 5′- or 3′-end-labelled oligonucleotides ( Supplementary Table S2 ) in binding buffer (5 × : 50 m M Tris-HCl, pH 7.5, 5 m M MgCl 2 , 2.5 m M EDTA, 2.5 m M dithiothreitol, 250 m M NaCl, 0.25 μg μl −1 poly(dI-dC):poly(dI-dC), 20% glycerol; Promega). The electrophoretic mobility shift binding assays were performed at room temperature for 30 min in the same buffer as for the nuclease assays, except with 10 mM EDTA. DNA–protein complexes and DNA products were separated on 10% native or 25% denaturing acrylamide gels, and PhosphorImager radiographs were quantified using ImageQuant software. Generation of polyclonal antibodies The 6 × His-MEIOB (245–466 aa) fusion protein was expressed in E. coli using the pQE-30 vector, affinity purified with Ni-NTA resin and used to immunize rabbits and guinea pigs (Cocalico Biologicals Inc.), yielding antisera UP2327 (rabbit) and UP-GP 99 (guinea pig). Affinity-purified antibodies were used for immunofluorescence and western blotting analyses. Other antibodies used for western blotting are ACTB (1:7,500, catalogue number A5441, clone AC-15, Sigma), histone H3 (1:2,500, catalogue number 05-499, clone 6.6.2, Millipore) and TEX19 (1:500) [13] . Targeted inactivation of the Meiob gene In the targeting construct, a 9-kb genomic DNA segment harbouring exons 6–10 of Meiob was replaced with the neomycin selection cassette ( Fig. 5a ). The two homologous arms (2.2 kb each) were amplified from a Meiob -containing BAC clone (RP23-397O23) by PCR with high-fidelity DNA polymerase. The thymidine kinase-negative selection marker was inserted adjacent to the right arm. V6.5 embryonic stem cells were electroporated with linearized pUP105/ClaI targeting construct, cultured in the presence of 350 μg ml −1 G418 and 2 μM ganciclovir and screened by long-distance PCR [12] . Out of 384 double-resistant embryonic stem cell clones, two homologously targeted clones were obtained and both yielded germline transmission of the Meiob mutant allele through chimeric mice. All offspring were genotyped by PCR. Wild-type allele (514 bp) was assayed by PCR with primers 5′-AGAGCCTTCTTTCACAATG-3′ and 5′-TTTATCTGCCCAGGACTAC-3′. The mutant allele (382 bp) was assayed by PCR with primers 5′-ACCTATACATTGGTGACCTTGA-3′ and 5′-CCTACCGGTGGATGTGGAATGTGTG-3′. Mice were maintained and used for experimentation according to the guidelines of the Institutional Care and Use Committee of the University of Pennsylvania. Statistics Statistical analysis was performed with Student’s t -test. The values were presented as mean±s.d. Histological and surface nuclear spread analyses For histological analysis, testes or ovaries were fixed in Bouin’s solution overnight, embedded with paraffin and sectioned using a microtome. Sections were processed and stained with haematoxylin and eosin. For immunofluorescence analysis, testes or ovaries were fixed in 4% paraformaldehyde for 3 h at 4 °C, dehydrated in 30% sucrose, processed and sectioned. TUNEL assays were carried out with the ApopTag Fluorescein In Situ Apoptosis Detection Kit (catalogue nunber S7110, Serologicals Corporation/Chemicon). For spread analysis, spermatocytes from postnatal day 16 testes were used unless noted otherwise. Testicular tubules or embryonic ovaries were extracted in a hypotonic treatment buffer. Cells were suspended in 0.1 M sucrose and were then spread on a thin layer of paraformaldehyde solution containing Triton X-100 (ref. 34 ). The following primary antibodies were used for immunofluorescence on spread nuclei: SYCP1 (1:50, catalogue number ab15090, Abcam), SYCP2 (ref. 12 ), SYCP3 (1:100, catalogue number 611230, BD Biosciences), γH2AX (1:500, catalogue number 16-202A, Clone JBW301, Millipore), ATR (1:200, catalogue number PC538, EMD Biosciences), RPA1 (1:50, catalogue number ab87272, Abcam), RPA2 (1:100, catalogue number 2208S, clone 4E4, Cell Signaling Technology), RAD51 (1:50, gift from late Peter Moens), DMC1 (1:50, catalogue number sc-22768 (H-100), Santa Cruz Biotech), MLH1 (1:50, catalogue number 550838, clone G168-15, BD Biosciences), MSH4 (1:50, gift from Chengtao Her) [53] , SPATA22 (1:50, catalogue number 16989-1-AP, ProteinTech Group) and TEX11 (1:10) [34] . Co-IP analysis Co-IP was performed with P18 testes using anti-MEIOB antibodies ( Fig. 7a ). Testes (200 mg) were homogenized in 1 ml RIPA buffer (50 mM Tris, pH 7.5, 150 mM NaCl, 1% NP-40, 1 mM dithiothreitol, 0.5% sodium deoxycholate, 0.05% SDS, 1 mM EDTA) with 1 × protease inhibitor cocktail III. Immunoprecipitated proteins were run on a 4–15% gradient SDS–PAGE gel and stained with SYPRO Ruby (Bio-Rad). The protein band exclusive to the wild-type testis sample was subjected to mass spectrometry. For co-IP experiments followed by western blotting ( Fig. 7b ), 200 mg of P18 testes (wild type or Meiob −/− ) were homogenized in 1 ml RIPA buffer plus 1 × protease inhibitor cocktail III on ice and 4 ml cold RIPA buffer with 1 × protease inhibitor cocktail III, and 90 U benzonase per ml was added to the lysate. The lysate was incubated on a rocking platform at room temperature for 2 h, followed by centrifugation at 16,100 g for 15 min at 4 °C. The supernatant was transferred to a new tube and centrifuged again at 100,000 g for 1 h at 4 °C. The supernatant was used for IP with anti-MEIOB antibodies followed by western blotting. Full scans of key western blottings are provided in Supplementary Fig. S12 . How to cite this article: Luo, M. et al. MEIOB exhibits single-stranded DNA-binding and exonuclease activities and is essential for meiotic recombination. Nat. Commun. 4:2788 doi: 10.1038/ncomms3788 (2013).